Cationic mononuclear ruthenium carboxylates as catalyst prototypes for self-induced hydrogenation of carboxylic acids Carboxylic acids are ubiquitous in bio-renewable and petrochemical sources of carbon. Hydrogenation of carboxylic acids to yield alcohols produces water as the only byproduct, and thus represents a possible next generation, sustainable method for the production of these alternative energy carriers/platform chemicals on a large scale. Reported herein are molecular insights into cationic mononuclear ruthenium carboxylates ([Ru(OCOR)] + ) as prototypical catalysts for the hydrogenation of carboxylic acids. The substrate-derived coordinated carboxylate was found to function initially as a proton acceptor for the heterolytic cleavage of dihydrogen, and subsequently also as an acceptor for the hydride from [Ru–H] + , which was generated in the first step (self-induced catalysis). The hydrogenation proceeded selectively and at high levels of functional group tolerance, a feature that is challenging to achieve with existing heterogeneous/homogeneous catalyst systems. These fundamental insights are expected to significantly benefit the future development of metal carboxylate-catalysed hydrogenation processes of bio-renewable resources. A great variety of carboxylic acids (CAs) is abundantly available from both the petrochemical industry and natural sources. The hydrogenation of CAs is an important research subject with respect to using the resulting alcohols as alternative organic energy (H 2 ) carriers, or as platform chemicals [1] . According to a 2004 report from the US Department of Energy, the vast majority of high value-added chemicals from biomass at that time were CAs [2] . While this number has been revised since, due to technological advancements, CAs remain prominent biomass products on this continuously changing list [3] . Alternatively, CAs can be generated synthetically, and an elegant synthesis was recently reported using CO 2 , H 2 and olefins [4] . Furthermore, formic acid has been produced by hydrogenation of CO 2 (refs 5 , 6 , 7 , 8 ), or by the photo-reduction of CO 2 with H 2 O using solar energy [9] . The availability of carbon-neutral alternatives to fossil fuels presents a critical challenge for the scientific community on the way to a more sustainable society. When CAs are sourced from biomass and/or produced from CO 2 , they represent a potential renewable resource. Finally, recent progress in C–H bond functionalization chemistry has demonstrated the versatility and utility of CAs as effective directing groups in organic synthesis [10] . The hydrogenation of CAs is an ideal method for the bulk production of alcohols, and may thus benefit the ‘methanol economy’, that is, the anthropogenic chemical carbon cycle [11] , [12] , since water is the only byproduct and salt waste is not formed. A hydrogenation method that is widely applicable to a broad variety of CAs and that selectively produces alcohols is therefore highly desirable. Unfortunately, however, simple molecular hydrogenation catalysts that enable such conversions still remain elusive. This is predominantly due to the lack of a rational design strategy for single-active-site catalysts that effectively hydrogenate the thermodynamically stable and kinetically inert COOH group in the absence of undesirable side reactions involving the COOH or other potentially present functional groups. In addition, the catalyst should be able to operate under acidic conditions, given the ex vi termini acidity of CAs. This is an important issue, since the catalytic hydrogenation of CA derivatives such as esters [13] , [14] , [15] and amides [14] , [15] , [16] proceeds well under basic to neutral conditions, but has seldomly been investigated when using a CA as the acidic reaction medium [15] . Even though conventional approaches to the hydrogenation of CAs with heterogeneous or homogeneous catalysts allow control over a number of reaction parameters, they usually proceed under fair to vigorous conditions ( P H2 =2.5–13 MPa and/or T =100–500 °C), and they frequently suffer from low alcohol selectivity/productivity [17] , [18] , [19] , [20] , [21] , [22] as a result of esterification (Ru 0 /Ru II ) [17] , [18] , [19] , partial reduction to afford aldehydes (Cr 2 O 3 ; ref. 20 ), over reduction (Re VII –Os VIII ; ref. 21 ), and/or dearomatic hydrogenation (Rh 0 –Mo 0 ; ref. 22 ). Even under milder conditions (typically: P H2 =2–3 MPa, T =120–130 °C), decarboxylation (Pt(–Re)/TiO 2 ; ref. 23 ) and esterification (Ir III or Rh III ; ref. 24 ) of some CAs represent significant shortcomings. Moreover, studies on functional group tolerance, which may provide useful information for organic synthesis have not yet been reported. In the presence of catalytic Brønsted acids and Ru–triphos complexes [25] , [26] , [27] , [28] , [29] , [30] , [31] , [32] (triphos=CH 3 C[CH 2 PPh 2 ] 3 ; Ph=C 6 H 5 ), a group of 4-oxo- and 4-hydroxy-CAs, including levulinic acid and succinic acid, undergoes hydrogenation under harsher conditions ( P H2 = ∼ 10 MPa, T = ∼ 200 °C) to afford alcohols [27] , [28] , [29] , [30] . Very recently, Leitner and co-workers [31] reported the [Ru(triphos)(TMM)]-catalysed (TMM=trimethylene methane) hydrogenation of acetic acid (AcOH; P H2 =6 MPa, T =180 °C), hexanoic acid and benzoic acid ( P H2 =5 MPa, T = ∼ 220 °C) (ref. 32 ) in the presence or absence of catalytic amounts of HN(SO 2 CF 3 ) 2 under relatively strenuous conditions. The corresponding alcohols were obtained in moderate to excellent yields (conversion of CAs: 50–99%). However, in many cases, this should be the result of in situ -generated esters (lactones) or anhydrides that serve as intermediates, which are able to undergo hydrogenation more effectively [26] , [27] , [28] , [29] , [30] , [31] , [32] , [33] , [34] . For instance, Ru–triphos complexes hydrogenate esters such as methyl benzoate and alkyl formates under milder conditions (for example, P H2 =3–5 MPa, T =140 °C) (refs 28 , 32 ). In addition, Goldberg and co-workers [24] demonstrated experimentally that CAs with shorter aliphatic carbon chains such as AcOH react much more rapidly, which is consistent with previous observations [17] , [18] , [19] . When the size of the CA increases from C 1 to C 4 , the corresponding carboxylate carbon atom becomes more electron rich and thus less susceptible to nucleophilic attack from transition metal hydrides. Herein, we would like to report a molecular prototype that benefits from the rational design for a single-active-site Ru catalyst for the hydrogenation of CAs [35] . The CA-derived carboxylate coordinated to the Ru centre was found to function initially as a proton acceptor in the heterolytic cleavage of dihydrogen, and subsequently also as a acceptor for a hydride from [Ru–H] + , which was generated in the first step. This catalytic cycle thus represents a CA self-induced CA hydrogenation. This catalyst affords the corresponding alcohols selectively and exhibits a high functional group tolerance. Conversely, the hydrogenation of esters is not promoted, and this catalytic system thus constitutes a benchmark achievement that may be potentially useful for selective organic synthesis and for the development of future catalytic hydrogenation methods for feedstock derived from biomass or CO 2 . Ruthenium carboxylates as catalyst prototypes Catalyst prototypes ( Fig. 1a ) for CA self-induced CA hydrogenation, and the characteristics of the present work that differ from earlier studies ( Fig. 1b ) are shown as the outline of this study. 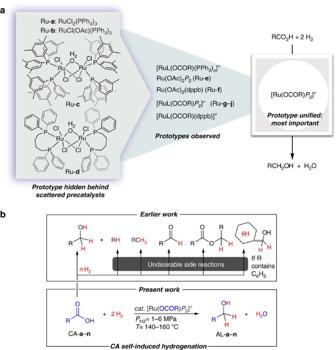Figure 1: Outline of this study. (a) The most favourable R is a saturated aliphatic group.P2denotes two monodentate or a bidentate phosphine ligand(s) and the search for optimalP2still remains the subject of further optimization. (b) CA self-induced CA hydrogenation (present work), in contrast to the shortcomings of earlier CA hydrogenation methods. Figure 1: Outline of this study. ( a ) The most favourable R is a saturated aliphatic group. P 2 denotes two monodentate or a bidentate phosphine ligand(s) and the search for optimal P 2 still remains the subject of further optimization. ( b ) CA self-induced CA hydrogenation (present work), in contrast to the shortcomings of earlier CA hydrogenation methods. Full size image Hydrogenation using Ru complex with monodentate phosphine Since the milestone discovery of the Wilkinson-type ruthenium complex RuCl 2 (PPh 3 ) 3 (Ru- a ) for the hydrogenation of olefins in the 1960s (refs 36 , 37 ), custom-tailored molecular single-active-site catalysts that hydrogenate CAs effectively have scarcely been investigated systematically [24] , [32] . The hydrogenation of 3-phenylpropionic acid (CA- a ; Table 1 , entry 1) in toluene using a combination of Ru- a (2 mol%: [Ru] 0 =6.7 mM), NaBPh 4 (10 mol%), and high pressure of H 2 ( P H2 =8 MPa, T =160 °C, t =24 h) resulted in the formation of alcohol AL- a and the ester Ph(CH 2 ) 2 CO 2 (CH 2 ) 3 Ph (ES- a ) in 58% and 16% yield, respectively (overall conversion of CA- a : 92%). In the absence of NaBPh 4 , Ru- a was unable to promote the hydrogenation, suggesting that a cationic Ru complex [L n Ru] + should be of critical importance for a successful hydrogenation. Instead of NaBPh 4 , other similar additives were tested, for example, NaB[3,5-(CF 3 ) 2 C 6 H 3 ] 4 , NaBF 4 , NaPF 6 , NaOTs, NaOTf and NaNTf 2 , but the results were unsatisfactory (AL- a : 0–17%). Encouraged by these results, several commercial derivatives of Ru- a , including RuCl 2 (PPh 3 ) 4 , RuHCl(CO)(PPh 3 ) 3 , RuCl 2 (CO) 2 (PPh 3 ) 2 , Ru( p -cymene)Cl 2 [P(C 6 H 11 ) 3 ], Ru(C 5 H 5 )Cl(PPh 3 ) 2 , cis -RuCl 2 (DMSO) 4 , and Ru(C 5 H 5 )Cl(dppm) (DMSO=dimethylsulfoxide; dppm=1,1-bis(diphenylphosphino)methane) were screened in the presence of NaBPh 4 (for details, see: Supplementary Table 1 ). However, the obtained yield of AL- a and ES- a was consistently below 10%. In contrast, the acetato complex RuCl(OAc)(PPh 3 ) 3 (Ru- b ; OAc=CH 3 CO 2 − ) afforded AL- a (55%) and ES- a (17%) in yields that were similar to those of Ru- a . Since a catalytic amount of the Ru-acetato complex Ru- b can readily undergo ligand exchange with excess CA- a in the reaction mixture, the general formula ‘[Ru(OCOR)] + ’ (R=aliphatic group) is assigned to the critical structure of the catalyst. Although H–H bond scission is known to be promoted by [Ru(OAc)] species [25] , [38] , [39] , [40] , investigations of their potential use have so far been focused more on the hydrogenation of unsaturated carbon–carbon bonds. Table 1 Hydrogenation of CAs using catalytic amounts of Ru- c , Ru- d or Ru- e . * Full size table To determine the best molar amount of PPh 3 relative to Ru sufficient to catalyse the hydrogenation of CA- a , the precatalyst was switched from Ru- a to RuCl 2 (DMSO) 4 (2 mol%, [Ru] 0 =6.7 mM) and varying molar amounts of the phosphine ligand was used in the presence of 10 mol% NaBPh 4 . The best results, which provided similar hydrogenation rates, were observed for a 2:1 and 3:1 ratio of PPh 3 and RuCl 2 (DMSO) 4 , while a 1:1 ratio significantly diminished the reaction rate. 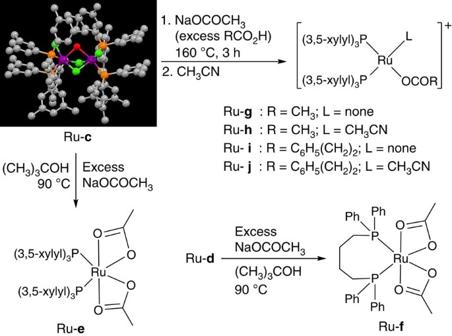Figure 2: Importance of ‘[Ru(OCOR)]+’ and its precursors for CA hydrogenation. Single crystal X-ray structure of Ru-c(containing ethanol). Colour code: Ru (purple), Cl (green), P (orange), O (red) and C (grey). Calculated exact masses: Ru-g(853.2872), Ru-h(894.3137), Ru-i(943.3341) and Ru-j(984.3607). From the thirteen different monodentate phosphines tested (for details, see: Supplementary Table 2 ), P(3,5-(CH 3 ) 2 (C 6 H 3 )) 3 (P(3,5-xylyl) 3 ) afforded the best yield (AL- a (ES- a ): 49% (14%)). To gain insight into the structural differences between the [Ru−P(3,5-xylyl) 3 ] complex and Ru- a , the synthesis of the corresponding Ru complex was attempted by treatment of RuCl 3 · n H 2 O with P(3,5-xylyl) 3 in a molar ratio of 1:6, following the experimental procedure reported for Ru- a [36] ( Supplementary Methods ). However, the expected Wilkinson-type 16e – complex Ru II Cl 2 (P(3,5-xylyl) 3 ) 3 was not obtained. Instead, the binuclear 18e – Ru complex Ru II 2 Cl 2 (μ-Cl) 2 (μ-OH 2 )(P(3,5-xylyl) 3 ) 4 (Ru- c ; see Figs 1a and 2 , wherein hydrogen atoms are omitted for clarity) was isolated as a reddish brown precipitate in 83% yield (for the X-ray crystallographic analysis, metric parameters, and an ORTEP structure of Ru- c , see: Supplementary Fig. 1 ). As a solid, Ru- c can be easily stored and handled, even under atmospheric conditions. Addition of a third phosphine ligand to the Ru centre, analogous to the formation of Ru- a proved to be impossible, presumably due to the sterically congested environment of Ru- c . This structural preference is consistent with the observation that a 2:1 ratio between the monodentate phosphine and Ru secured efficient catalysis. When using Ru- c (1 mol%) with NaBPh 4 (10 mol%), hydrogenation of CA- a proceeded more effectively, even under a lower hydrogen pressure ( P H2 =4 MPa), affording AL- a and ES- a in 65 and 12% yield, respectively ( T =160 °C, t =24 h; conversion of CA- a : 92%). 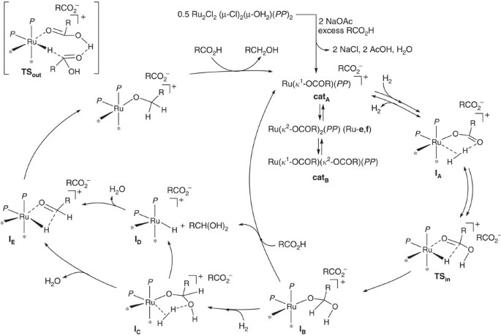Figure 3: Plausible catalytic cycle involving ‘[Ru(OCOR)P2]+’. P2denotes 2P(3,5-xylyl)3or dppb. The asterisk (*) denotes various neutral ligands including solvents such as toluene or dioxane. Replacing NaBPh 4 with NaOAc and Na(acac; acac=acetylacetonate) resulted in comparable effectiveness, furnishing AL- a (ES- a ) in 62% (15%) and 64% (14%) yield, respectively ( Supplementary Table 3 ). Figure 2: Importance of ‘[Ru(OCOR)] + ’ and its precursors for CA hydrogenation. Single crystal X-ray structure of Ru- c (containing ethanol). Colour code: Ru (purple), Cl (green), P (orange), O (red) and C (grey). Calculated exact masses: Ru- g (853.2872), Ru- h (894.3137), Ru- i (943.3341) and Ru- j (984.3607). Full size image The reaction conditions were further optimized by slightly increasing the load of Ru- c to 1.5 mol% so that the hydrogenation was accelerated relative to the simultaneously occurring in situ esterification. Furthermore, the more atom-economical NaOAc (10 mol%) was used as the additive for the hydrogenation of various CAs ( P H2 =2–4 MPa, T =140–160 °C). The results are given in Table 1 ( Supplementary Methods for representative methods). Aliphatic acids CA- b and CA- c were hydrogenated chemoselectively, exclusively producing alcohols AL- b and AL- c (entries 2 and 4). This contrasts with the heterogeneous Pt–Re/TiO 2 -catalysed hydrogenation system, in which the decarboxylation of CA- c predominates, affording the by one carbon atom diminished alkane [23] . As CA- d , was sterically the most demanding CA, we expected it to be kinetically the most inert. Indeed for the hydrogenation of CA- d , a slower reaction rate was observed, but AL- d was generated cleanly and esterification was not observed (entry 5). CA- e (α-phenoxy acid) was one of the most reactive CAs tested, and hydrogenation proceeded smoothly even under relatively mild conditions ( P H2 =2 MPa, T =140 °C; entry 6). When the hydrogenation of CA- e with Ru- c (1.5 mol%) and NaOAc (10 mol%) was stopped after 6 h (AL- e : 50%), more than 90% of free AcOH (based on added NaOAc) were detected by 1 H NMR. This result suggests the exclusive formation of a [Ru(OCOCH 2 OPh)] + species, which does not promote the hydrogenation of AcOH, but should be responsible for hydrogenation of CA- e (that is, a CA- e self-induced CA- e hydrogenation). This is in agreement with the previously discussed result, which proposed a [Ru(OCOR)] + complex derived from Ru- b as the active catalyst. In contrast, benzoic acid CA- l was one of the least reactive substrates (entry 15). And indeed, with the exception of one very recent example [32] , the chemoselective hydrogenation of arenyl (Ar) CAs (ArCO 2 H) using molecular catalysts has so far failed. For instance, both the benzene ring and the carboxyl group of CA- l are fully hydrogenated using Rh/Al 2 O 3 –Mo(CO) 6 as the catalyst system [22] . Relative to aliphatic carboxylates, arenyl carboxylates ( – OCOAr) such as those derived from CA- l should be more strongly coordinated to Ru complexes in a κ 2 -manner [41] , [42] . The nature of the more favourable κ 2 -complexation prevents [Ru(OCOAr)] + from forming a [Ru(η 2 -H 2 )] + species, since the coordination sites of Ru are effectively occupied, rendering the electrophilicity of the Ru centre too low to trap the σ H–H bond. Subsequent formation of a ruthenium hydride, bearing the protonated carboxylate, [RuH(HOCOR)] + , is also more favourable with an aliphatic group than with aryl group, that is, the intramolecular deprotonation of η 2 -H 2 should proceed more readily in the κ 1 -carboxylate structure [Ru(η 2 -H 2 )(κ 1 -OCOR)] + than in the κ 2 -carboxylate, where the carboxylate (R≠Ar) is more basic and thus a less innocent ligand [38] , [39] , [40] , [41] , [42] , [43] , [44] . Indeed, the hydrogenation of CA- a in three different initial concentrations ([CA- a ] 0 =200, 333 and 500 mM) was consistently more sluggish in the presence of a small amount of CA- l ([CA- l ] 0 =67 mM; CA- l :Ru- c =13:1) than in the absence of CA- l , and it also afforded AL- a consistently in lower yields. However, irrespective of the presence ( t =2.5 h) or absence ( t =1.5 or 2.5 h) of CA- l , the reaction rates obtained with the three different initial concentrations [CA- a ] 0 in each series were roughly equivalent, providing approximately the same [AL- a ] t =2.5 (0.06–0.09 M with CA- l versus 0.08–0.11 M without CA- l . For the dependence of different [CA- a ] 0 with the same [CA- l ] 0 on yields of AL- a and AL- l , see: Supplementary Fig. 2 ). The hydrogenation rate was observed to be virtually independent of [CA- a ] 0 , whereby the initially added CA- l was recovered effectively (CA- l : 78–99%; AL- l : 5–10%) in all three runs. These results suggested that the catalytic hydrogenation giving AL- l promoted by [Ru(OCOPh)] + via an inner-sphere mechanism was barely involved. The catalysis facilitated by the more reactive [Ru(OCO(CH 2 ) 2 Ph)] + via an outer-sphere mechanism (cleavage of H–H bond, followed by an intermolecular hydride transfer from the resulting [RuH(HOCO(CH 2 ) 2 Ph)] + to a free CA- l ) was also negligible. These processes scarcely interfere with the faster catalysis mediated by [Ru(OCO(CH 2 ) 2 Ph)] + or [RuH(HOCO(CH 2 ) 2 Ph)] + that affords AL- a (CA- a self-induced CA- a hydrogenation in the presence of CA- l ). To reconfirm that indeed the suspected ‘CA self-induced CA hydrogenation’ was observed here, the hydrogenation of CA- l was also carried out using three different initial concentrations ( t =6 h). As in the previous case, a zeroth order rate with respect to [CA- l ] corroborates a CA- l self-induced CA- l hydrogenation ( Supplementary Fig. 3 ). These preliminary kinetic experiments indicated that the apparent reaction rate of CA hydrogenation with Ru- c and NaOAc at the same parameters for [H 2 ] and T is independent of [CA] t and almost constant, assuming a constant [[Ru(OCOR)] + ] t . In other words, the velocity of the rate-determining step should change only on varying the concentration of [Ru(OCOR)] + . It is therefore suggested that CA- a and CA- l should be involved not only as integral ‘carboxylates’ of the catalysts for cleaving the H–H bond, but also as ‘protonated carboxylates’ that are spontaneously activated and reduced by the resulting [Ru–H] + , which is generated in the first step of the CA self-induced CA hydrogenation. The CO 2 H groups of CA- h and CA- i were hydrogenated more rapidly than the interior aliphatic and aromatic esters, furnishing AL- h and AL- i chemoselectively, under preservation of the methyl ester moieties (entries 10 and 12). In addition, when a 1:1 molar mixture of CA- d and ethyl stearate (CH 3 (CH 2 ) 16 CO 2 CH 2 CH 3 ) was hydrogenated using Ru- c (1.5 mol%) and NaOAc (10 mol%; P H2 =4 MPa, T =160 °C, t =24 h), AL- d was obtained in 99% yield, while the ester was recovered unchanged. An external ester did not inhibit the catalysis and did not engage with the [RuH(HOCOR)] + species (R=1-adamantyl). The [RuH(HOCOR)] + complex should be accessible only by a CA covalently attached to the Ru centre. In contrast, esters that cannot covalently bind to the Ru complex may have little chance to participate in the catalytic cycle as an integral structure of the catalyst. The applied conditions are most likely not basic enough to effectively promote the homocoupling of alcohols, and therefore the occurrence of a Tishchenko-type reaction giving esters can be excluded ( Supplementary Methods ). Moreover, it seems that the condensation of the CA with the alcohol to give the corresponding ester is also effectively suppressed in the present system, since the catalyst is unable to hydrogenate esters. The benzene rings in close proximity to or spatially removed from the CA groups of CA- a , e , f , i , j and CA- l–n were well tolerated (entries 1, 6–8, 12, 13 and 15–18), whereas the amide moiety of CA- f (entry 7) and the thiophene moiety of CA- g (entry 9) inhibited the catalysis. Despite the fact that the olefin moieties of CA- i – k were hydrogenated (entries 12–14), the high chemoselectivity and concurrent compatibility of aromatic rings and ester moieties achieved here is virtually unprecedented and rarely achieved with typical, strong, stoichiometric agents such as LiAlH 4 , LiBH 4 , BH 3 or LiBEt 3 H that reduce not only CAs, but also esters [45] . Hydrogenation using Ru complex with bidentate phosphine To improve the catalytic activity, the combination of a multidentate ligand (2 mol%), RuCl 2 (DMSO) 4 (2 mol%) and NaBPh 4 (10 mol%) was examined in detail. From a variety of multidentate ligands screened ( Supplementary Table 2 ), 1,4-(diphenylphosphino)butane (dppb) proved to be one of the best (AL- a : 52%, ES- a : 14%; P H2 =8 MPa, T =160 °C, t =24 h). Another elegant approach that differs from ours was reported by Leitner and Klankermayer, who proposed [Ru(triphos)(OCOH)] + and Ru(triphos)(TMM) species as the catalytically active species for the hydrogenation of CO 2 ( P H2 =5 MPa, T =140 °C) and CA- l ( P H2 =50 bar, T =220 °C) (ref. 32 ), giving CH 3 OH (ref. 31 ) and AL- l , respectively. Nevertheless, RuCl 2 (DMSO) 4 /triphos (2 mol% each) was observed to be less effective for CAs with a longer carbon chain (AL- a : 22%, ES- a : 13%). Moreover, the catalyst systems Ru(acac) 3 /triphos (2 mol% each) [26] , [30] and [Ru(triphos)(TMM)] (refs 31 , 32 ) (2 mol%) were tested separately ( P H2 =8 MPa, T =160 °C, t =24 h), but the observed reactivity was consistently low (AL- a : 22% and 10%, ES- a : 10% and 8%, respectively). In contrast, it became clear that a [Ru(dppb)] complex could adopt a structure Ru- d [46] , which is similar to Ru- c . Hence, Ru- d (1 mol%) with Na(acac) (10 mol%) was tested for the hydrogenation of CA- a ( P H2 =4 MPa, T =160 °C, t =24 h), which furnished an improved yield of 78 and 10% for AL- a and ES- a , respectively, under almost quantitative conversion of CA- a . Using Ru- d , it was also possible to hydrogenate the relatively unreactive substrate CA- l under much milder conditions than those reported by Leitner [32] , affording AL- l in 93% yield ( Table 1 , entry 16). The increased catalytic activity of Ru- d relative to that of Ru- c could also be demonstrated by the following experiment: Ru- c and Ru- d (1.5 mol% each) were used separately with Na(acac) (10 mol%) for the hydrogenation of CA- l ( P H2 =4 MPa, T =160 °C, t =48 h), giving AL- l in 26% and 56%, respectively (benzyl benzoate: 2% and 1%, respectively). Substrates CA- m and CA- n , carrying electron-donating and -withdrawing groups, respectively, were also compatible with these conditions ( Table 1 , entries 17 and 18). Moreover, the hydrogenation of other substrates that were relatively inert to the Ru- c /NaOAc system also proceeded more readily when using Ru- d and Na(acac; Table 1 , entries 3 and 11). Another advantage of Ru- d over Ru- c is the structural robustness of the catalyst derived from Ru- d under aqueous conditions ( Supplementary Table 4 ). Insight into catalytic [Ru(OCOR) P 2 ] + The prospective resting state of these catalysts, a [Ru(OCOR) P 2 ] + species, was elucidated by electrospray ionization-mass spectroscopy (ESI–MS) analysis ( Fig. 2 and Supplementary Figs 4 and 5 ). After a toluene solution of a 1:6.7 mixture of Ru- c and NaOAc was heated to 160 °C for 3 h, a sample thereof was dissolved in MeCN and examined by ESI–MS, which revealed two primary signals ( m / z =853.2856 and 894.3137) corresponding to Ru- g and Ru- h , respectively. Presumably, the catalytically innocent species [RuH(CO)[P(3,5-xylyl) 3 ] 2 ] + ( m / z =823.2752, exact mass: 823.2766) was observed, as its parent compound Ru(OAc)H(CO)[P(3,5-xylyl) 3 ] 2 could be detected by 31 P{ 1 H} NMR in CDCl 3 (δ 45.8 (s, P RuP) and 45.9 (s, PRu P ) p.p.m. (ref. 47 ). When a toluene solution of a 1:6.7:33 mixture of Ru- c , NaOAc and CA- a was heated to 160 °C for 3 h, Ru- i , Ru- j and Ru- h were detected as the primary signals ( m / z =943.3291, 984.3645 and 894.3083, respectively). In both ESI–MS measurements, binuclear structures (involving two Ru centres) could not be detected. The catalytically important structure ‘[Ru(OCOR) P 2 ] + ’, consistent with Ru- i and Ru- j , could not be obtained in significant amounts when NaB[3,5-(CF 3 ) 2 C 6 H 3 ] 4 , NaBF 4 , NaOTf or NaNTf 2 were used as additives instead of NaOAc or NaBPh 4 ( Supplementary Figs 6 and 7 ). One of the original Cl − groups of Ru- c remained unaffected, or was replaced by CO. In addition, after a (CH 3 ) 3 COH solution of a 1:20 mixture of Ru- c and NaOAc was heated to 90 °C for 2 h, Ru- e was isolated in 49% yield ( Fig. 2 ; Supplementary Methods ). The hydrogenation of CA- a with Ru- e (3 mol%, [Ru] 0 =10 mM) proceeded effectively ( P H2 =4 MPa, T =160 °C, t =24 h) in the absence of NaOAc, giving AL- a (ES- a ) in 87% (6%) yield, which is comparable to previously obtained results. In the absence of NaOAc (under less basic conditions) and using a small amount of dioxane (10 equiv with respect to CA- a ), esterification was more effectively suppressed ( Table 1 , entry 8). Using Ru- e , the α,β-unsaturated aliphatic CA tiglic acid (CA- k ) was hydrogenated at both the olefin and the CO 2 H groups, giving 2-methyl-1-butanol (AL- k ) in ca. 65% yield ( Table 1 , entry 14). We would like to use this opportunity to underline the unique reactivity of our system relative to previously described systems: using the comparable Ru-acetato complex Ru(CO) 2 (OCOCH 3 ) 2 (PBu 3 ) 2 (Bu=CH 3 (CH 2 ) 3 ) did not lead to the hydrogenation of the CO 2 H groups of CA- k or 2-methylbutanoic acid ( P H2 =ca. 13 MPa, T =100 °C) [19] . Here the CA self-induced CA hydrogenation via the cationic mononuclear complexes [Ru(OCOR)] + was not observed and the hydrogenation of AcOH was ascribed to ‘unknown catalytic species’, affording the ester AcOCH 2 CH 3 . A higher catalytic activity of binuclear Ru-carboxylato complexes relative to that of mononuclear derivatives [18] , [19] and the importance of intermediary Ru(acyl)(alkoxy) complexes were briefly discussed [18] . The Ru-diacetato complex Ru- f was synthesized from Ru- d ( Fig. 2 ) [48] and was one of the most active Ru catalysts for the hydrogenation of CA- a under relatively mild conditions ( P H2 =2 MPa; Table 2 ), even though a slightly decreased yield of AL- a was observed under lower hydrogen pressure ( P H2 =1 MPa; entry 5). In contrast, hydrogenation with Ru- e proceeded comparably, but more selectively using a lower [CA- a ] 0 (entry 3 versus 4). The high alcohol selectivity should be ascribed, at least partially, to the low [CA] 0 . Table 2 Comparison experiments using the Ru(OAc) 2 P 2 complexes Ru- c and Ru- d under lower hydrogen pressure ( P H2 =1–2 MPa) for the hydrogenation of CA- a . * Full size table On the basis of these observations, we would like to propose a catalytic cycle ( Fig. 3 ). Figure 3: Plausible catalytic cycle involving ‘[Ru(OCOR) P 2 ] + ’. P 2 denotes 2P(3,5-xylyl) 3 or dppb. The asterisk (*) denotes various neutral ligands including solvents such as toluene or dioxane. Full size image Important points that corroborate the catalytic cycle can be summarized as: (1) Ru-dicarboxylates such as Ru- e and Ru- f are stable enough to be isolated; (2) NaBPh 4 (replacing Cl − in Ru- c or Ru- d to generate the catalytically active cationic Ru complex) as well as NaOAc effective induced the catalyst; (3) the rate of the hydrogenation was effectively decreased when using Ru- e ( P H2 =4 MPa, T =160 °C, t =24 h) in dioxane as a solvent (AL- a : 60%; ES- a : 2%), which strongly coordinates to the cationic Ru centre; (4) although Ru(CO) complexes were detected by ESI–MS ( vide supra ), the attachment of CO to the Ru centres should be excluded from the catalytic cycle, since such a coordination of CO would be detrimental to the catalytic activity of the CA hydrogenation under mild conditions; and (5) the intermediate ‘[RuH(dppb)] + ’, corresponding to I D or I E stabilized by toluene ( m/z found: 621.1425, calcd: 621.1409) or by CH 3 CN ( m/z found: 570.1047, calcd: 570.1048) was observed in addition to a [Ru(OCOR)(dppb)] + species analogous to Ru- i and Ru- j . Those species were generated by treatment of a toluene solution of Ru- f with CA- a and H 2 (Ru- f :CA- a (mol%)=1:33, [CA- a ] 0 =333 mM, P H2 =4 MPa, T =160 °C, t =3 h) and were detected in CH 3 CN solution by ESI–MS analysis (for all Ru species observed, see: Supplementary Fig. 8 ). Another critical intermediate identified was 18e − η 6 -toluene-stabilized I B [Ru(OCH(OH)(CH 2 ) 2 Ph)(dppb)(toluene)] + ( m/z found: 771.2001, calcd: 771.2089). Moreover, [Ru[OCO(CH 2 ) 2 Ph](dppb)(CH 3 CN)] + [ m/z found: 718.1601 (the strongest intensity), calcd: 718.1572] as stabilized cat A is consistent with the unified ‘prototype [Ru(OCOR) P 2 ] + ’ in the catalytic cycle involving the CA self-induced CA hydrogenation ( I A → TS in → I B ). By taking these facts into account, a cationic ruthenium complex cat A incorporating one carboxylate is likely the most critical and active species, although catalysis involving the two carboxylate-bearing cat B can not be fully ruled out. Since the hydrogenation rate using Ru- e was affected by the H 2 pressure (1–4 MPa; Supplementary Fig. 9 ), the formation of Ru–η 1 -H ( TS in ) via Ru–η 2 -H 2 complex I A should be the turnover-limiting step in this P H2 range. A multifunctional (outer sphere) mechanism ( TS out ; Fig. 3 ) involving a RCO 2 – moeity [49] and a RCO 2 H molecule (with a cooperative role for RuH(δ – ) and Ru[H(δ + )OCOR] for hydrogen transfer to another RCO 2 H), as an alternative to a TS in (inner-sphere mechanism involving direct interaction of the CA with a Ru centre; Fig. 3 ), might be also possible, although an unambiguous assignment requires a further detailed kinetic and theoretical analysis. Even though free aldehydes were not detected, the release of free hemiacetal from I C via a four-centered σ-bond metathesis giving I D , or through the hemiacetal–CA exchange of I B that affords cat A , followed by dehydrative formation of free aldehyde that re-enters the catalytic cycle to give I E , is another possible scenario. In any case, further refinement of the molecular design of CA hydrogenation catalysts based on the catalytic cycle proposed involves two key factors: (1) the formation of a Ru–η 1 -H species through deprotonation of the Ru–η 2 -H 2 is facilitated by the participation of a cationic [Ru(OCOR)] + (R=aliphatic group) species. This step may involve a pathway analogous to the concerted metalation–deprotonation mechanism proposed for the cleavage of either H–H (refs 25 , 38 , 39 , 40 , 49 ) or C–H bonds [41] , [42] , [43] , [44] . (2) The CA reformed via the protonation of Ru-carboxylate remains coordinated to the cationic Ru centre of Ru–H species ( I A → TS in ). This activated CA in TS in is more electrophilic and should be able to facilitate a smooth hydride transfer from the Ru–H species to the carbonyl carbon atom. In summary, the results obtained from the systematic study of these cationic, mononuclear ruthenium mono-carboxylate catalyst prototypes enabled a rational approach to the design of hydrogenation catalysts for CAs. The results demonstrate that the CAs should act not only as integral carboxylates for the catalysts to cleave the H–H bond, but also as protonated carboxylates that are simultaneously activated and reduced by the resulting [Ru–H] + , which is generated in the first step (CA-induced CA hydrogenation). As the availability of bidentate phosphines is virtually infinite, further optimization of the ligand for better catalyst performance under milder conditions is ongoing, together with an extension of the present fundamental research, which has provided this milestone discovery. Identification of ideal metal carboxylates that hydrogenate bio-renewable resources in high oxidation states will significantly benefit the future development of chemical processes directed towards a sustainable society. Accession codes : The X-ray crystallographic coordinate for the structure (Ru- c ) reported in this Article has been deposited at the Cambridge Crystallographic Data Centre (CCDC), under deposition number CCDC 1024070. The data can be obtained free of charge from The Cambridge Crystallographic Data Centre via www.ccdc.cam.ac.uk/data_request/cif . How to cite this article: Naruto, M. et al. Cationic mononuclear ruthenium carboxylates as catalyst prototypes for self-induced hydrogenation of carboxylic acids. Nat. Commun. 6:8140 doi: 10.1038/ncomms9140 (2015).